Correspondence: Reply to ‘Reassessing the contribution of natural gas to US CO2emission reductions since 2007’ 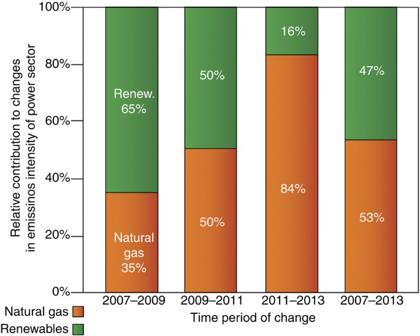Figure 1 Relative contributions of natural gas and renewables to the changes in emissions intensity of US power sector. How to cite this article: Feng, K. et al . Correspondence: Reply to ‘Reassessing the contribution of natural gas to US CO 2 emission reductions since 2007’. Nat. Commun . 7:10693 doi: 10.1038/ncomms10693 (2016).